Viscoelastic solids explain spider web stickiness Modern orb-weaving spiders have evolved well-designed adhesives to capture preys. This adhesive is laid on a pair of axial silk fibres as micron-sized glue droplets that are composed of an aqueous coat of salts surrounding nodules made of glycoproteins. In this study, we measure the adhesive forces required to separate a small microscopic probe after bringing it in contact with a single glue droplet. These forces are highly rate-dependent and are two orders of magnitude higher than the capillary forces. The glycoproteins in the glue droplets behave as a viscoelastic solid and the elasticity is critical in enhancing adhesion caused by specific adhesive ligands. These results have important implications in mimicking bioadhesives. Nature has evolved a myriad of well-designed adhesives that assist in locomotion, self-defence and prey capture. Geckos use micron-sized hairs as dry adhesives for locomotion. Mussels secrete specialized proteins to stick under water. Modern orb-weaving spiders use micron-sized glue droplets laid on a pair of viscoelastic axial silk for catching prey [1] . These glue droplets are composed of granules of glycoproteins surrounded by viscous aqueous coats of salts that regulate water content [2] , [3] , [4] . Many attempts to understand the nature of these adhesives and to mimic their properties emphasize on determining the ligands in the glycoproteins responsible for adhesion, but ignore critical aspects of the structure itself. This is partly because of an inability to probe the glycoproteins through the viscous coat and partly because of the difficulty in separating the contribution of the glue droplets from the highly extensible axial silk for the force required to peel a single thread off a surface [5] . Here, by directly probing single adhesive droplets used by spiders, we demonstrate the importance of the mechanics of adhesive in dramatically enhancing adhesion. We show that glue drops function as a viscoelastic material instead of as a viscous material and that the elasticity of the principle adhesive in this system, the glycoproteins, increases adhesion by two orders of magnitude in comparison with capillary forces, thus putting to rest the old notion of the adhesive being viscous. Glycoproteins behave as a viscoelastic solid—a property that has important consequences in increasing the stickiness of these almost invisible capture silk threads. At slow extension rates, similar to the movements of trapped insects, glycoproteins deform like an ideal elastic rubber band, which is essential in retaining the insects trapped in the web long enough to be subdued by the spider. At high extension rates, the adhesive forces are dramatically enhanced because of high viscous effects, making it easier for the capture silk threads to hold on to fast-flying insects when they initially impact webs. Exhibition of similar adhesion strategies in these distinct species (geckos, mussels and spiders) suggests a common design principle in the evolution of natural adhesives [6] . These results emphasize that the structure and mechanics of these adhesives are important in enhancing the adhesive forces. 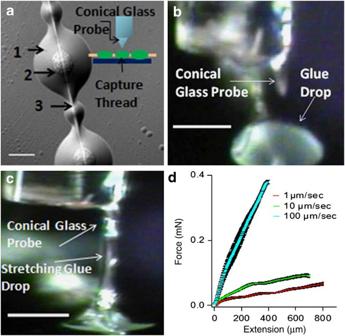Figure 1: Single glue drop adhesion measurements. (a) The components of the capture thread of the spiderL. cornutus:(1) viscous coat, (2) glycoprotein granule and (3) axial thread. Scale bar is 20 μm. Recently, it has been suggested that the viscous coat contains transparent layers of glycoproteins8. Inset shows a schematic of the single drop pulling experiments, wherein single glue drops (green) of a capture thread were stretched using a conical glass probe (blue) while force responses were recorded. (b) The conical glass probe approaching a single glue drop. Scale bar is 50 μm. (c) Stretching of a single glue drop using the conical glass probe. Scale bar is 60 μm. (d) Force responses when single glue drops were stretched at different rates until separation from the glass probe. Curves are plotted as mean ± s.d. from three measurements each (error bars are in black for all three cases). Measurement of capillary forces Capture silk threads are immobilized on a glass substrate and a conical glass probe of 10 μm base diameter is brought into contact with glue droplets as shown in Figure 1a,b . The probe is then retracted at constant speeds ( Fig. 1c ) while the force is recorded as a function of distance ( Fig. 1d ). After reaching the critical pull-off force, the tip releases contact. The visual image of glue droplets stretching is shown in Figure 1c . The force–distance response is highly dependent on the rate of pull-off. Pull-off forces increase from 60 μN at a rate of 1 μm s −1 to around 400 μN at 100 μm s −1 ( Fig. 1d ). Figure 1: Single glue drop adhesion measurements. ( a ) The components of the capture thread of the spider L. cornutus: (1) viscous coat, (2) glycoprotein granule and (3) axial thread. Scale bar is 20 μm. Recently, it has been suggested that the viscous coat contains transparent layers of glycoproteins [8] . Inset shows a schematic of the single drop pulling experiments, wherein single glue drops (green) of a capture thread were stretched using a conical glass probe (blue) while force responses were recorded. ( b ) The conical glass probe approaching a single glue drop. Scale bar is 50 μm. ( c ) Stretching of a single glue drop using the conical glass probe. Scale bar is 60 μm. ( d ) Force responses when single glue drops were stretched at different rates until separation from the glass probe. Curves are plotted as mean ± s.d. from three measurements each (error bars are in black for all three cases). Full size image To rule out that pull-off forces are due to capillary effects, we measure capillary effect-induced pull-off forces by dipping the conical probe in a model polymeric viscous liquid (unentangled polydimethylsiloxane (PDMS), because it has high affinity for glass). These pull-off forces are below the detectable limit of the instrument (1 μN). Therefore, we use a larger diameter probe (90 μm) to measure the capillary effect-induced pull-off forces and then estimate the capillary forces for a 10 μm diameter probe using the Wilhelmy equation ( f c = γ × perimeter × cos Θ ). These estimates for PDMS ( γ ∼ 20 mN m −1 ) and a liquid of surface tension 40 mN m −1 (typical values expected for aqueous solutions such as viscous coat) are 0.6 and 1.3 μN, respectively (green and black markers in Fig. 2a ). The pull-off forces exerted by the glue droplets are two to three orders higher than the capillary forces, indicating that the primary adhesive in the system is the glycoprotein and not the viscous coat. 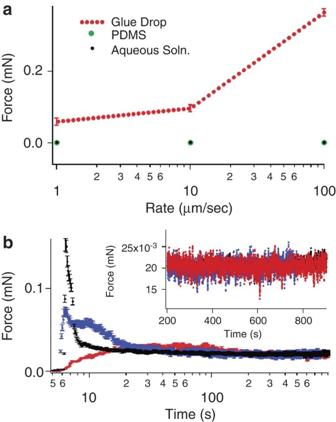Figure 2: Elasticity governs adhesion rather than capillary forces. (a) Compares the pull-off forces at different stretching rates for glue drops (red markers) with the capillary forces exerted by PDMS melt (Mw=6000 Da,Me=8000 Da,γ=19.8 mN m−1, green markers) and the calculated capillary forces exerted by the viscous coat (γ=40 mN m−1). For PDMS glass and viscous coat glass, the contact angleΘwas taken as 0. Values are plotted as mean ± s.d. from three measurements each. (b) Load-relaxation curves in which glue drops were stretched by 100 μm at three different rates (100 μm s−1(black), 10 μm s−1(blue), 1 μm s−1(red)), after which the load was allowed to relax. Inset shows an enlarged view of the plateau regions for the three cases. All measurements were taken close to 25 °C at 40% relative humidity (RH). The curves are plotted as mean ± s.d. from three measurements each. Figure 2: Elasticity governs adhesion rather than capillary forces. ( a ) Compares the pull-off forces at different stretching rates for glue drops (red markers) with the capillary forces exerted by PDMS melt ( M w =6000 Da, M e =8000 Da, γ =19.8 mN m −1 , green markers) and the calculated capillary forces exerted by the viscous coat ( γ =40 mN m −1 ). For PDMS glass and viscous coat glass, the contact angle Θ was taken as 0. Values are plotted as mean ± s.d. from three measurements each. ( b ) Load-relaxation curves in which glue drops were stretched by 100 μm at three different rates (100 μm s −1 (black), 10 μm s −1 (blue), 1 μm s −1 (red)), after which the load was allowed to relax. Inset shows an enlarged view of the plateau regions for the three cases. All measurements were taken close to 25 °C at 40% relative humidity (RH). The curves are plotted as mean ± s.d. from three measurements each. Full size image Viscoelasticity On the basis of the rate-dependence of pull-off forces, the glue could be either a viscoelastic liquid or a viscoelastic solid. If the glue is a viscoelastic liquid, then the glue should behave as a liquid at very low velocities. In contrast, if the glue is a viscoelastic solid, then forces will not relax to zero with time. To test these predictions, we measured the force-relaxation after stretching the glue droplets by 100 μm ( Fig. 2b ). For high speeds, there is considerable overshoot; however, with time, the forces relax to a constant value that is independent of the rate of displacement. The steady state forces, which are two orders of magnitude higher than those expected for capillary forces, clearly indicate that the glue is responding neither as a viscous liquid nor as a viscoelastic liquid. Instead, the glue exhibits characteristics of a viscoelastic solid. This is consistent with the microscopy images of a glycoprotein granule (and the whole glue drop) swelling in water while retaining its shape at high humidity ( Fig. 3a,b ). Furthermore, the elastic response and the absence of terminal flow regions indicate that the glycoproteins are physically or chemically crosslinked. 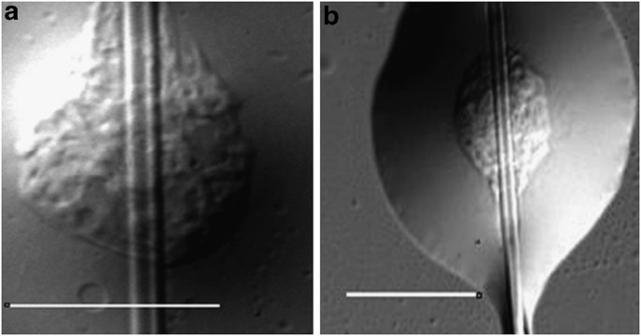Figure 3: Swelling of glue droplets at high humidity. (a,b) Transmission mode images of glycoprotein granules at 90 and 0% RH, respectively. Scale bars are 20 μm. Figure 3: Swelling of glue droplets at high humidity. ( a , b ) Transmission mode images of glycoprotein granules at 90 and 0% RH, respectively. Scale bars are 20 μm. Full size image Viscoelasticity of glue drops has far-reaching consequences on the functioning of capture threads in spider webs. A single capture thread is covered with many of these glue drops and the peeling of a capture silk thread from a surface depends on both glue drops and the viscoelasticity of silk fibres. 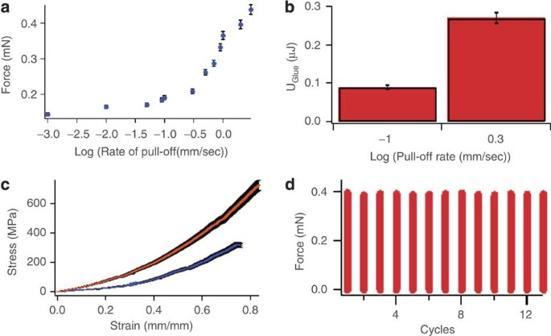Figure 4: Peeling capture silk thread from the surface depends on the peeling rate. (a) The effect of the rate of pull-off (dh/dt) on the force at pull-off (blue markers and black error bars). Values are plotted as mean ± s.d. from 15 measurements each. (b) Adhesion energies at two pull-off rates using the model explained in the text. (c) The stress–strain behaviour of capture spiral thread at the rate of 2 mm s−1(red) and 0.1 mm s−1(blue). The curves are plotted as mean ± s.d. from five measurements each. Error bars are in black for both cases. Measurements were taken at 40% RH close to 25 °C. (d) Repeatability of the force at pull-off of a capture thread ofL. cornutus. Measurements were taken close to 25 °C at 40% RH. The pull-off rate was 2 mm s−1. Figure 4a (blue markers) shows the force required to peel off a capture silk thread from a glass substrate at different rates. These peeling forces are reversible over many cycles ( Fig. 4d ). Interestingly, the peeling forces for whole threads depend on the rate, similar to the results we obtained for the pull-off forces of a single glue droplet. Because peeling forces depend on the mechanical properties of both silk fibres and the glue, we need to separate the contributions of each component. Figure 4: Peeling capture silk thread from the surface depends on the peeling rate. ( a ) The effect of the rate of pull-off (d h /d t ) on the force at pull-off (blue markers and black error bars). Values are plotted as mean ± s.d. from 15 measurements each. ( b ) Adhesion energies at two pull-off rates using the model explained in the text. ( c ) The stress–strain behaviour of capture spiral thread at the rate of 2 mm s −1 (red) and 0.1 mm s −1 (blue). The curves are plotted as mean ± s.d. from five measurements each. Error bars are in black for both cases. Measurements were taken at 40% RH close to 25 °C. ( d ) Repeatability of the force at pull-off of a capture thread of L. cornutus . Measurements were taken close to 25 °C at 40% RH. The pull-off rate was 2 mm s −1 . Full size image The work performed to pull a silk thread off a surface is consumed in stretching of the axial silk and the energy required to peel glue droplets from the surface. 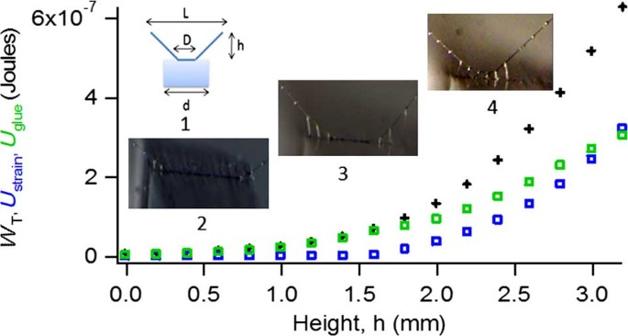Figure 5: Model to separate the adhesive energy from the strain energy stored in silk fibres. The geometry used for the pull-off measurements is shown in inset 1. The total work (black) carried out in separating the thread from the surface, strain energy stored in the axial silk (blue), and the energy contribution of the glue drops (green) when the thread went through the consecutive stages shown as insets 2, 3 and 4. Calculation ofUstrainandUglueinvolved the reasonable approximation thatD≪L. In these experiments, this condition is satisfied (0 mm ≤D≤ 2 mm andL=16 mm). The final values ofUstrainandUgluedo not depend on the condition thatD≪L. Figure 5 (inset 1) shows a sketch defining the variables used in the energy model. The total work on the system ( W T ) is calculated by integrating the product of the force f(h) times the infinitesimal height change d h from h to h +d h . Figure 5: Model to separate the adhesive energy from the strain energy stored in silk fibres. The geometry used for the pull-off measurements is shown in inset 1. The total work (black) carried out in separating the thread from the surface, strain energy stored in the axial silk (blue), and the energy contribution of the glue drops (green) when the thread went through the consecutive stages shown as insets 2, 3 and 4. Calculation of U strain and U glue involved the reasonable approximation that D ≪ L . In these experiments, this condition is satisfied (0 mm ≤ D ≤ 2 mm and L =16 mm). The final values of U strain and U glue do not depend on the condition that D ≪ L . Full size image The strain energy stored in the thread when it is pulled from its initial position until it separates from the surface, U strain , is given by the following equation: σ ( ɛ ) is the value of stress at strain, ɛ and r are the radii of the thread. Stress–strain characteristics of the silk thread depend on the rate of deformation and are shown in Figure 4c . Subtracting Equation (2) from Equation (1) gives the energy required to separate the glue drops from the surface, U glue . The values of U glue depend on intermolecular adhesion, as well as on the energy required to stretch the glue droplets. The contributions of U glue and U strain are shown in Figure 5 for a peeling experiment at a rate of 2 mm s −1 . Using this energy model, we determine the values of U glue for 0.1 and 2 mm s −1 peeling rates ( Fig. 4b ). Similar to single drop experiments, the peeling of the silk thread from the surface is also rate dependent and is strongly coupled with the elasticity of the glue droplets. We can now compare the work performed by the glue droplets obtained from peeling experiments versus single glue droplet measurements. The area under the load-displacement curve ( Fig. 1d ) corresponds to the energy required to pull off the glass fibre after probing the glue droplet. On the basis of the distance of ∼ 40 μm between the centres of the two droplets, we estimate that there are 42 large glue droplets in a 2 mm length thread. Multiplying the work performed by one glue droplet by the total number of drops, we estimate the upper limit of U glue (1, 1.4 and 3.4 μJ at rates of 1, 10 and 100 μm s −1 , respectively). However, individual glue droplets neither stretch at constant rates nor to the same extent during peeling experiments. Furthermore, the surface area of the probe used for single drop measurement is larger than the area of contact between single glue droplets and the substrate during a thread peeling experiment. These factors lead us to conclude that energy values determined from the single droplet measurements define the upper limit of U glue . Most importantly, the rate dependence of U glue observed in these experiments illustrates that the viscoelastic properties of the glue have an important role in the adhesion of capture silk threads and their ability to capture prey. In summary, we show here that glycoproteins in orb-weaving spider capture silk use elasticity to enhance their adhesive forces during prey capture. Although there is no direct evidence of the molecular nature of the glue's elasticity, a recent study demonstrates that one of the glycoproteins in Nephila clavipes capture silk has amino-acid sequences similar to elastin and flagelliform spider silk and may therefore possess some level of elasticity [7] . These results suggest that one of the strongest bioadhesives known to mankind evolved an intricate composition that consists of not only glycosylated and chitin adhesive groups [7] but also an elastic backbone. Marine mussels also use elasticity to enhance the adhesive forces of their byssal threads [6] . We conclude that the mechanical properties of the adhesive have a major role in determining adhesion and that designing a successful mimic of a biological adhesive requires understanding both the ligand responsible for adhesion and the elasticity of the backbone structure. Single drop pulling Capture threads from orb webs spun by Lariniodes cornutus were immobilized on a glass slide. Measurements of adhesion were taken using an MTS Nano Bionix that measured force to ± 1 μN. The glass slide was fixed firmly on the lower clamp, whereas a clean conical glass probe (base diameter=10 μm) was fixed on the upper clamp. To measure adhesion, the conical probe was lowered at 1 μm s −1 till it made firm contact with a glue drop (the whole assembly was observed with an optical microscope). After 60 s, the probe was pulled away from the silk at known rates. The stretching behaviour of the glue drop was observed using an optical microscope, simultaneously recording the load-displacement response every 0.01 s. Capillary measurements Polydimethylsiloxane of viscosity 100 cSt (obtained from Gelest Inc.) was filled in a pan of diameter 8 mm and depth 3 mm, which was fixed firmly on the lower clamp of the Nano Bionix. A cylindrical glass probe of diameter 90 μm, fixed on the top clamp, was dipped in the PDMS at a rate of 1 μm s −1 , held there for 60 s and then retracted at known rates. The load-displacement response was recorded every 0.01 s. Thread pull-off measurements Individual fibres of capture spiral silk were first collected from the webs spun by Larinioides cornutus and adhered to cardboard mounts across 16 mm gaps. After mounting the sample in the Nano Bionix, we pressed the silk thread onto a 2 mm-wide piece of glass mounted on a small tack. The glass was replaced regularly so that every run was performed on a clean surface. The sample was first lowered until it initially contacted the glass, and then pressed until the force registered 80 μN to ensure firm contact. Finally, the silk was pulled away from the substrate at known rates. Stickiness was measured directly as the force registered when the silk released from the substrate. Confocal microscopy To observe swelling of glue droplets, individual threads were equilibrated at a desired humidity. After equilibration, the threads were pressed onto a coverslip so that the force registered was 80 μN. The coverslip was covered with another coverslip quickly and the edges were then sealed to maintain the targeted humidity. Images were then taken using an Olympus IX71 with a ×100 objective. How to cite this article: Sahni, V. et al . Viscoelastic solids explain spider web stickiness. Nat. Commun. 1:19 doi: 10.1038/ncomms1019 (2010).